Caution in inferring viral strategies from abundance correlations in marine metagenomes 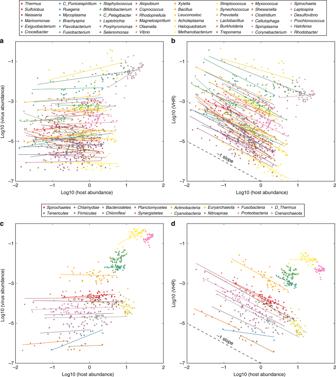Fig. 1 Relationships between virus abundances, virus–host ratios (VHRs), and host abundances.aGenus-level relationships, virus vs. host abundances.bGenus-level relationships, VHRs vs. host abundances.cPhylum-level relationships, virus vs. host abundances.dPhylum-level relationships, VHRs vs. host abundances. Panelsbanddare replotted from ref.1. The absence of a relationship between original, untransformed virus and host abundances (see panelsaandc) should appear as a −1 slope when comparing VHR to host abundances (see panelsbandd). A −1 slope is shown as a guide to readers in panelsbandd 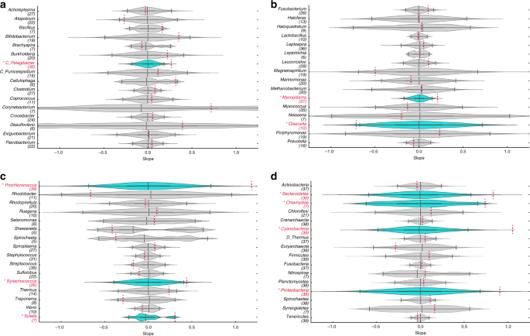Fig. 2 Violin plots of the 95% randomized confidence intervals (CIs) of the slope for relationships between virus and host abundances.a–cCIs in genus datasets.dCIs in phylym datasets. In each panel, red dashed lines indicate the slope of the original sample. Dark vertical lines indicate the 2.5, 50, and 97.5 percentiles. Datasets with slopes withp≥ 0.05 are shown in gray violin plots and datasets with slopes withp< 0.05 are shown in blue violin plots. The number of data points for each dataset is indicated in the parenthesis below the genus/phylum name Datasets The datasets of Coutinho et al. [1] were partitioned based on whether interactions were identified at the genus or phylum scale. In the original dataset, there were 17 and 93 virus–host datasets at the phylum scale and genus scale respectively. Each dataset has 39 distinct sampling sites. However, those sites with zero virus abundance or zero host abundance were excluded. In addition, we did not include any datasets for which there were not at least five sample sites with both non-zero levels of microbes and viruses. As a result, the datasets analyzed included 16 of 17 original virus–host pairs at the phylum level and 48 of 93 original virus–host pairs at the genus level. Statistical analysis We implemented permutation tests to assess measured correlations between virus and host abundances. For each host dataset we generated 10 4 randomized samples of size n i (the number of sample sites for virus–host pair i ). In each sample, we permuted the virus abundances without replacement while holding the host abundances fixed. Distributions of measured correlations were compared to the original samples using product–moment correlation (main text and Supplementary Information) and Spearman rank correlation (see Supplementary Information).